Differentiated availability of geochemical mercury pools controls methylmercury levels in estuarine sediment and biota Neurotoxic methylmercury (MeHg) formed from inorganic divalent mercury (Hg II ) accumulates in aquatic biota and remains at high levels worldwide. It is poorly understood to what extent different geochemical Hg pools contribute to these levels. Here we report quantitative data on MeHg formation and bioaccumulation, in mesocosm water-sediment model ecosystems, using five Hg II and MeHg isotope tracers simulating recent Hg inputs to the water phase and Hg stored in sediment as bound to natural organic matter or as metacinnabar. Calculations for an estuarine ecosystem suggest that the chemical speciation of Hg II solid/adsorbed phases control the sediment Hg pool’s contribution to MeHg, but that input of MeHg from terrestrial and atmospheric sources bioaccumulates to a substantially greater extent than MeHg formed in situ in sediment. Our findings emphasize the importance of MeHg loadings from catchment runoff to MeHg content in estuarine biota and we suggest that this contribution has been underestimated. Methylmercury (MeHg) accumulated in estuarine fish is a major concern for wildlife and human health [1] . It may originate from direct atmospheric and terrestrial MeHg loading or may form in estuaries from inorganic divalent Hg (Hg II ) [2] , [3] , [4] . Also Hg II is deposited to estuaries from the atmosphere or runoff and partly accumulates over time in sediment as various solid and adsorbed chemical forms [1] . The extent to which these different geochemical MeHg and Hg II pools, a term that we here define as Hg with different chemical speciation and/or environmental compartment localization, contribute to MeHg in sediment and biota is largely unknown [5] . Improved knowledge is critical for our understanding of the Hg biogeochemical cycle, to manage Hg pollutant issues and to predict the impact of changes in Hg emission rates, climate and anthropogenic land use. Formation of MeHg is a biotic process carried out by specific strains of sulphate- and iron-reducing bacteria, methanogens and firmicutes [4] , [6] , [7] , [8] , and mediated via the hgcA and hgcB genes [7] . Such bacteria have been suggested to take up and methylate specific aqueous Hg II -complexes, that is, neutral Hg II sulphide [3] (although recently questioned [9] , [10] ) or low-molecular-mass Hg II thiol complexes [11] , [12] . Only a minor fraction of Hg II in natural sediment and waters is present in the aqueous phase, and the partitioning to the solid phase (K D ) is typically in the range 10 5 −10 6 l kg −1 (ref. 13 ). To sustain typically observed methylation rates, aqueous concentrations of Hg II must continuously be resupplied by dissolution/desorption from the much more abundant solid/adsorbed Hg II phases [14] . We recently showed, using small-scale sediment slurry experiments, that the Hg II methylation rate constant ( k m ) differed up to 2 orders of magnitude depending on the Hg II solid phase speciation [14] . In addition to factors controlling MeHg formation, concentration of MeHg in biota is influenced by factors regulating the entry of MeHg into the food web and its trophic transfer. Irrespective of whether the cellular uptake mechanisms involve dissolved MeHg complexes in surrounding water or in the gut, the uptake is governed by the chemical speciation of dissolved MeHg and to a large extent limited by sorption to particles or complexation with dissolved organic ligands, which are not bioavailable [15] , [16] , [17] . Yet our understanding of processes controlling the availability of different geochemical MeHg pools, and the quantitative importance of such processes at the ecosystem level, remains insufficient. Generation of quantitative data on the availability for MeHg formation and bioaccumulation of specific geochemical Hg pools relevant for ecosystem level models requires experimental systems that represent natural conditions with respect to factors critical for MeHg formation (that is, natural sediment redox gradients, relevant bacterial community structure and a continuous supply of autochthonous organic carbon to the benthic zone) and bioaccumulation (relevant pelagic and benthic food webs). The experimental procedure is thus challenging, however, by the use of a new mesocosm experimental setup enabling the study of model ecosystems with intact sediment cores, and combining it with a recently developed isotope tracer methodology [14] , we were able to meet these requirements. We show that the solid/adsorbed phase chemical speciation of Hg II in the sediment and catchment runoff loading rate of MeHg are the major factors controlling MeHg quantity in estuarine sediment and biota. The contribution to MeHg in sediment and biota from long-term accumulated Hg pools in sediment is controlled by the solid/adsorbed phase chemical speciation of Hg, where Hg II bonded to thiol groups in natural organic matter (NOM) is ten times more available for methylation than metacinnabar (β-HgS). Further, recent inputs of MeHg from terrestrial runoff (or to a minor extent from atmospheric deposition) exhibit a 5–250 times higher availability for bioaccumulation as compared with MeHg formed in situ in the sediment. We propose that the contribution of MeHg loadings from catchment runoff to MeHg content in estuarine biota has, in many systems, been underestimated. Mesocosm experimental system and Hg isotope tracers Model ecosystems with intact sediment cores (~0.2 × 0.63 m Ø) submerged in brackish water were constructed in high-density polyethylene (HDPE) cylinder mesocosms ( n =3, 2,000 l volume, 5 m × 0.75 m Ø) and controlled with respect to temperature, light exposure and nutrient additions during an experimental period of 2 months. Isotopically enriched Hg II and MeHg tracers were injected across the sediment cores (surface injection density of 1.1 injection per cm 2 and injection depth of 0.5 cm) as solid/adsorbed chemical forms relevant for suboxic/anoxic conditions [14] (metacinnabar: β- 200 HgS sed and complexes with thiol groups in NOM: 201 Hg II -NOM sed and Me 198 Hg-NOM sed ) to simulate accumulated sediment Hg II and MeHg pools. A second set of tracers were added to the brackish water as labile aqueous Hg II and MeHg complexes ( 204 Hg II wt and Me 199 Hg wt ) to simulate recent Hg inputs to the water phase (from atmospheric deposition and catchment runoff), see Fig. 1 . The MeHg/Hg II molar ratio ( Supplementary Methods , Supplementary Fig. 1 ) determined in sediment samples was used as a quantitative measure of the rate of net MeHg formation ( Fig. 2a,b ) and remained fairly stable from the second week of the experiment. Bioaccumulation of MeHg in plankton (seston size fractions), amphipods and benthic invertebrates collected at the end of the experiment was quantified by the Biota-Sediment Accumulation Factor (BSAF; MeHg concentration ratio between biota (pmol g −1 dry weight (d.w.)) and sediment (pmol g −1 d.w.; Fig. 2c–e ). 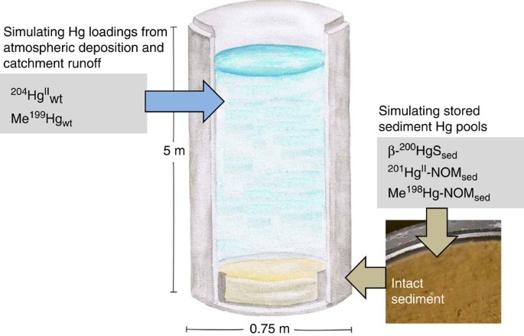Figure 1: Illustration of the experimental setup. Schematic illustration of the Hg isotope tracer addition and representation in the mesocosm systems. Figure 1: Illustration of the experimental setup. Schematic illustration of the Hg isotope tracer addition and representation in the mesocosm systems. 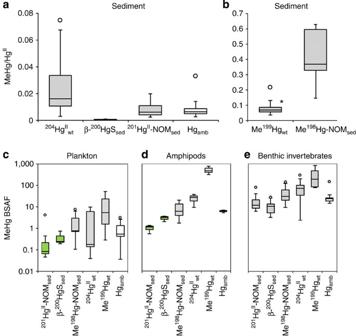Figure 2: MeHg/HgIImolar ratio and MeHg Biota-Sediment Accumulation Factor (BSAF). Box plots showing 25th, 50th and 75th percentiles (horizontal bars), 1.5 interquartile ranges (error bars) and maximum outlier (open circles) for MeHg/HgIImolar ratio determined in mesocosm sediment samples from days 10 to 52 of the experiment for (a) HgIItracers and ambient Hg (white bar) and (b) MeHg tracers. Asterisk indicates calculated minimum ratio for Me199Hgwtbased on a theoretical [HgII] value if 100% of the tracer had deposited to the sediment. Corresponding box plots for BSAF of MeHg from HgIIand MeHg tracers and ambient MeHg (white bars) in (c) plankton (seston size fractions 50–100, 100–300 and >300 μm), (d) amphipods and (e) benthic invertebrates (Chironomids,Polychaetesand bivalves) collected at the end of the experiment (day 57). Green coloured boxes indicate limit of detection data. Full size image Figure 2: MeHg/Hg II molar ratio and MeHg Biota-Sediment Accumulation Factor (BSAF). Box plots showing 25th, 50th and 75th percentiles (horizontal bars), 1.5 interquartile ranges (error bars) and maximum outlier (open circles) for MeHg/Hg II molar ratio determined in mesocosm sediment samples from days 10 to 52 of the experiment for ( a ) Hg II tracers and ambient Hg (white bar) and ( b ) MeHg tracers. Asterisk indicates calculated minimum ratio for Me 199 Hg wt based on a theoretical [Hg II ] value if 100% of the tracer had deposited to the sediment. Corresponding box plots for BSAF of MeHg from Hg II and MeHg tracers and ambient MeHg (white bars) in ( c ) plankton (seston size fractions 50–100, 100–300 and >300 μm), ( d ) amphipods and ( e ) benthic invertebrates ( Chironomids , Polychaetes and bivalves) collected at the end of the experiment (day 57). Green coloured boxes indicate limit of detection data. Full size image MeHg net formation Net MeHg formation (average MeHg/Hg II ±confidence interval (CI), p =0.05) of the 201 Hg II -NOM sed tracer (0.0084±0.0025) was higher (14–18 times) than of the β- 200 HgS sed tracer (0.00049±0.00013; Fig. 2a ). This result is in line with our previous small-scale experiments [14] and reasonable given the low solubility of β-HgS(s) [10] . Further, we observed a MeHg/Hg II ratio for 204 Hg II wt (0.027±0.012) that was 3–4 and 40–70 times higher than for 201 Hg II -NOM sed and β- 200 HgS sed , respectively ( Fig. 2a ). Separate incubation experiments with tracer-spiked mesocosm water (which remained oxic throughout the entire experiment) showed that MeHg formation in the water phase was negligible. We thus conclude that the 204 Hg II wt tracer was methylated in the sediment. The average residence time of this tracer in the water column was 10–15 days ( Supplementary Fig. 2a ), which highly exceeds the time of ~10 h to maximum a few days [18] , [19] typically needed for Hg II to rearrange from its predominant labile Hg(OH) 2 0 complex to the thermodynamically most stable NOM coordinated complexes. Under the existing oxic conditions in the DOC-rich water column, a coordination with two thiols (RSH): Hg(SR) 2 in NOM would be the by far dominant complex [20] ( Supplementary Table 1 ). Therefore, the 204 Hg II wt tracer should have depostited to the sediment as Hg(SR-NOM) 2 complexes either after flocculation/aggregation of NOM and/or after adsorption to water column particles [21] . Based on this argumentation, we regard the 204 Hg II wt tracer to be representative of Hg II recently deposited from the atmosphere and from terrestrial runoff. It cannot be ruled out that differences in the character of NOM in the water column of the mescocoms (a mixture of allochthonous and autochthonous NOM to which 204 Hg II wt can be expected to complex) and the pure terrestrial NOM used in the 201 Hg II -NOM sed tracer are important for the higher MeHg/Hg II ratio observed for the 204 Hg II wt tracer. This is, however, not likely given that terrestrial NOM constitutes more than 75% of the total DOC in the estuary where the mesocosm brackish water was collected [22] . It also needs to be considered that the 204 Hg II wt tracer deposited to the surface of the sediment during an extended time of the experiment, whereas 201 Hg II -NOM sed was injected at a sediment depth of 0.5 cm at the start of the experiment. The pore water chemistry and bacterial activity usually change drastically with depth close to the surface in natural sediments [23] . In separate experiments, k m values determined in sediment slurries (from 4 cm Ø sediment cores sub-sampled from the mesocosms) were fairly constant (0.017–0.023 d −1 ) in the top 4 cm (1 cm resolution) and did thus not support vertical discrepancy to explain the differences in net MeHg formation. It may, however, be that the resolution (1-cm layers) was not fine enough to encapture the commonly encountered high rate of Hg II methylation in the sediment–water interface. Our results contribute to clarify the critical but uncertain question if recent Hg II deposits to the ecosystem water phase are more available for methylation than previous Hg deposits accumulated in the system [24] , [25] ( Figs 2a and 3a ). Our data support such a hypothesis but also shows that as a general statement this would be too simplistic. Depending on the chemical speciation of Hg II , the difference can be large (40–70 times) or relatively small (3–4 times) if the sediment pool is dominated by β-HgS(s) or by Hg(SR-NOM) 2 . 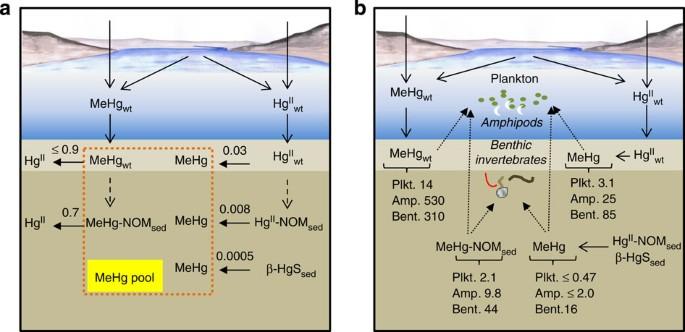Figure 3: Illustration of net formation and bioaccumulation of MeHg from different geochemical Hg pools. (a) Net formation (from HgIItracers) and net degradation (from MeHg tracers) of MeHg in sediment (0–1.5 cm) from stored sediment pools of HgII(HgII-NOMsed, β-HgSsed) and MeHg (MeHg-NOMsed) and from recent HgII(HgIIwt) and MeHg (MeHgwt) loadings to the aquatic system via atmospheric deposition or terrestrial runoff deposited to the sediment surface. Values are given as MeHg/HgIImolar ratio for HgIItracers and HgII/(HgII+MeHg) molar ratio for MeHg tracers. (b) Biota-Sediment Accumulation Factor for MeHg originating from the different HgIIand MeHg tracers for plankton (Plkt., average of 50–100, 100–300, >300 μm seston size fractions), amphipods (Amp.) and benthic invertebrates (Bent., average forChironomids,Polychaetesand bivalves). Figure 3: Illustration of net formation and bioaccumulation of MeHg from different geochemical Hg pools. ( a ) Net formation (from Hg II tracers) and net degradation (from MeHg tracers) of MeHg in sediment (0–1.5 cm) from stored sediment pools of Hg II (Hg II -NOM sed , β-HgS sed ) and MeHg (MeHg-NOM sed ) and from recent Hg II (Hg II wt ) and MeHg (MeHg wt ) loadings to the aquatic system via atmospheric deposition or terrestrial runoff deposited to the sediment surface. Values are given as MeHg/Hg II molar ratio for Hg II tracers and Hg II /(Hg II +MeHg) molar ratio for MeHg tracers. ( b ) Biota-Sediment Accumulation Factor for MeHg originating from the different Hg II and MeHg tracers for plankton (Plkt., average of 50–100, 100–300, >300 μm seston size fractions), amphipods (Amp.) and benthic invertebrates (Bent., average for Chironomids , Polychaetes and bivalves). Full size image MeHg degradation Based on previous incubation experiments [24] , [26] with dissolved labile isotope tracers (and assuming pseudo-first order rate laws for formation and degradation of MeHg), half-life (ln 2/ k d , where k d is the MeHg demethylation rate constant) and turnover ( k m + k d ) −1 of MeHg in natural sediments have been estimated to be on the order of 1–3 days. Based on this, the MeHg molecule has been considered not to persist or accumulate in natural sediments. Vertical sediment profiles have in some cases demonstrated a close correlation between MeHg concentration and the Hg II methylation rate [27] , in line with the hypothesis of a rapid MeHg turnover, whereas other studies have indicated that MeHg might persist longer (up to decades) in sediments [28] , [29] . If assuming 1–3 days turnover, the Me 198 Hg-NOM sed tracer would within ~2 weeks adopt a similar MeHg/Hg II ratio as our added Hg II tracers and ambient Hg in the mesocosm sediment. In great contrast, we observed a MeHg/Hg II ratio for Me 198 Hg-NOM sed that was on average 16–880 and 50 times higher than for Hg II tracers and ambient Hg, respectively, during the 52 days experiment ( Fig. 2a,b ). This observation indicates a much longer turnover, at least for a significant fraction of MeHg in sediments. Marvin-Dipasquale et al . [30] suggested that MeHg can be sequestered into several pools with different availability for demethylation. The fraction (approximately 30% if the remaining fraction is assumed to turnover in 1–3 days) of the Me 198 Hg-NOM sed tracer that was not readily available for demethylation in our study was still somewhat more efficiently bioaccumulated than MeHg formed in situ from the 201 Hg II -NOM sed and β- 200 HgS sed tracers ( Figs 2c–e and 3b ). We suggest that sequestration of MeHg as thermodynamically stable forms, such as complexes with thiols in NOM (or possibly adsorbed to sulphide minerals), in the sediment partly prevents demethylation yet without preventing MeHg entering the aquatic food webs. The exact mechanisms leading to the accumulation of persistent MeHg in sediments are, however, not well understood and their potential importance not well recognized. MeHg bioaccumulation We observed a considerably higher (5–250 times) BSAF for Me 199 Hg wt ( Figs 2c–e and 3b ), as compared with Me 198 Hg-NOM sed and in situ formed MeHg, in both plankton and benthic invertebrates. This, as well as our modelling results discussed below, clearly emphasizes the importance of imported MeHg for its bioaccumulation in estuarine ecosystems. This MeHg import will consist of a small proportion from direct atmospheric deposition and a large proportion from terrestrial runoff (originating from methylation of atmospherically depositied Hg II in catchment soils). Although direct input of MeHg is highly available for bioaccumulation, in situ formed MeHg (from atmospheric and runoff Hg II inputs) is bioaccumulated to a lower extent. We propose that this difference in bioaccumulation is mainly a consequence of feeding strategies of specific organisms [31] , [32] and differences in the vertical distribution of MeHg originating from different sources (in our case tracers). The Me 199 Hg wt tracer settles to the oxic sediment surface predominantly as MeHg, whereas for the other tracers, MeHg is formed (or for the Me 198 Hg-NOM sed tracer directly injected) in suboxic/anoxic zones a few millimetre below the sediment surface. The Me 199 Hg wt tracer will thus have the highest relative MeHg abundance in both the pelage (where zooplankton feed) and at the surface of the sediment. Amphipods and the benthic invertebrate species present in this study predominately feed on freshly deposited material at the water–sediment interface [31] . The time required for MeHg to establish its most thermodynamic stable configuration with NOM, as a one-coordinated MeHgSR complex [20] , is expected to be faster than the time required for the two-coordinated Hg(SR) 2 complex to form (discussed above). We therefore propose that MeHgSR–NOM complexes controlled the speciation of the Me 199 Hg wt tracer ( Supplementary Table 1 ) during the vast majority of its average residence time of ~7 days ( Supplementary Fig. 3a ) in the water column and that it settled to the sediment predominantly as such complexes. This explanation model is further supported by the fact that the MeHg Biota Accumulation Factor (l g −1 d.w., calculated as the average MeHg concentration in plankton divided by the average concentration in water from day 15) in plankton for the Me 199 Hg wt (54 l g −1 d.w) and ambient MeHg (23 l g −1 d.w; the only pools with detectable MeHg concentration in water) exhibited a smaller difference (factor of 2) than did BSAF (factor of 17) for Me 199 Hg wt (14) and ambient MeHg (0.8). This indicate that there was likely no significant difference in chemical speciation or availability of Me 199 Hg and ambient MeHg dissolved in the water column, but that a larger fraction of MeHg from the Me 199 Hg wt tracer was distributed to the water column and the sediment–water interface as compared with ambient MeHg, and likely also the other Hg tracers. Mercury mass balance modelling In this work, we provide the first quantitative data demonstrating how geochemical pools of Hg II and MeHg differ with respect to their availability for MeHg formation/degradation ( Fig. 3a ) and bioaccumulation ( Fig. 3b ). We evaluated to what extent these differences control MeHg concentrations in sediment and biota for estuarine ecosystems. Briefly, we applied the determined MeHg/Hg II ratios and BSAFs ( Fig. 3 ) and estimated pool sizes and fluxes of Hg II and MeHg for the Öre Estuary ( Table 1 ) in a simple mass balance model (equations (1) and (2)). Four scenarios, differing in Hg II solid/adsorbed phase speciation (scenario A1 and A2) or MeHg and Hg II loading rates (scenario A1, B and C), were postulated. These models exhibit qualitative features recognized as critical, but hitherto not included, in Hg biogeochemical modelling. Table 1 Estimated Hg deposition rates to sediment surface from specific flux sources and sizes of stored Hg sediment pools used in model scenarios A–C. Full size table It is evident that because of differentiated availability for MeHg formation and bioaccumulation, specific Hg pools are predicted to contribute differently to MeHg concentration in sediment and biota ( Fig. 4 ). The solid/adsorbed phase chemical speciation of Hg II in the sediment is a major controlling factor for MeHg levels in sediment and biota. As illustrated by scenarios A1 and A2, a [β-HgS]:[Hg II -NOM] molar ratio in the sediment of 30:70 compared with 70:30 would, for the same total sediment Hg II concentration, almost double the total amount of MeHg in the sediment and increase MeHg levels in biota by approximately 15–50%. The ‘persistent’ MeHg pool (purple bars in Fig. 4 ) is predicted to largely contribute to MeHg in sediment and biota for all the postulated scenarios. Further research is warranted to clarify if the build-up of this pool in sediments is simply a result of formation of thermodynamically stable MeHg–NOM complexes or if additional processes control the size of this pool. 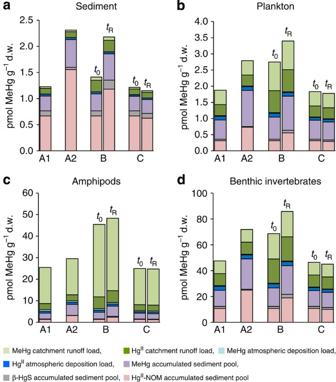Figure 4: Modelled contribution from different geochemical Hg pools to MeHg in sediment and biota. Predicted contributions from the seven HgIIand MeHg pools to MeHg concentrations in (a) 0–1.5 cm sediment layer, (b) plankton, (c) amphipods and (d) benthic invertebrates. The MeHg concentrations were calculated using equations (1) and (2) with the input data inTable 1and the MeHg/HgIImolar ratios and BSAFs determined from HgIIand MeHg isotope tracers in the mesocosm experiment (Fig. 3), estimated loading rates of HgIIand MeHg from catchment runoff and the atmosphere to the Öre Estuary, sizes of sediment pools for HgIIdetermined from average concentration of ambient HgIIfrom five sites within the estuary and for MeHg (XA1–C) calculated as 30% of the estimated sum concentration (pmol MeHg per g d.w.) of the other five contributing sources for each scenario (described in Supplementary Information). Scenario A1 estimated present day input fluxes to the Öre Estuary (described in Supplementary Information) and a β-HgS(s)/HgII-NOM molar ratio of 70:30 in sediment as determined by HgIILIII-edge EXAFS14; scenario A2: β-HgS(s)/HgII-NOM molar ratio of 30:70; scenario B: two times increase in catchment runoff loading compared with present day modelled for a time period of 4 months (t0) and the time period to replenish the Hg content in the 0–1.5 cm surface sediment (tR=15 years); scenario C: 27% decrease in total atmospheric HgIIloading compared with present day (reflecting a 40% decrease in anthropogenic atmospheric Hg emissions assumed to constitute two-third of the total atmospheric Hg emissions) modelled for a time period of 4 months (t0) and the time period to replenish the Hg content in the 0–1.5 cm surface sediment (tR). Figure 4: Modelled contribution from different geochemical Hg pools to MeHg in sediment and biota. Predicted contributions from the seven Hg II and MeHg pools to MeHg concentrations in ( a ) 0–1.5 cm sediment layer, ( b ) plankton, ( c ) amphipods and ( d ) benthic invertebrates. The MeHg concentrations were calculated using equations (1) and (2) with the input data in Table 1 and the MeHg/Hg II molar ratios and BSAFs determined from Hg II and MeHg isotope tracers in the mesocosm experiment ( Fig. 3 ), estimated loading rates of Hg II and MeHg from catchment runoff and the atmosphere to the Öre Estuary, sizes of sediment pools for Hg II determined from average concentration of ambient Hg II from five sites within the estuary and for MeHg (X A1–C ) calculated as 30% of the estimated sum concentration (pmol MeHg per g d.w.) of the other five contributing sources for each scenario (described in Supplementary Information). Scenario A1 estimated present day input fluxes to the Öre Estuary (described in Supplementary Information) and a β-HgS(s)/Hg II -NOM molar ratio of 70:30 in sediment as determined by Hg II L III -edge EXAFS [14] ; scenario A2: β-HgS(s)/Hg II -NOM molar ratio of 30:70; scenario B: two times increase in catchment runoff loading compared with present day modelled for a time period of 4 months ( t 0 ) and the time period to replenish the Hg content in the 0–1.5 cm surface sediment ( t R =15 years); scenario C: 27% decrease in total atmospheric Hg II loading compared with present day (reflecting a 40% decrease in anthropogenic atmospheric Hg emissions assumed to constitute two-third of the total atmospheric Hg emissions) modelled for a time period of 4 months ( t 0 ) and the time period to replenish the Hg content in the 0–1.5 cm surface sediment ( t R ). Full size image Comparing scenario B to A1, coupled with the findings of others [33] , [34] , suggest that MeHg levels in sediment and biota in estuarine ecosystems could be highly sensitive to variations in catchment runoff. We modelled the effect of a twofold increase in Hg II +MeHg runoff loading, which, for the Öre Estuary, predicts a rapid increase of MeHg in biota by 40–80% (t 0 , scenario B) and a 80–90% increase when the sediment layer simulated as active for MeHg formation and bioaccumulation in our model (0–1.5 cm) is fully replenished ( t R , scenario B). These results further emphasize the potentially large negative effects on MeHg levels in estuarine biota caused by increased terrestrial runoff following, for example, climate change-induced increases in precipitation or permafrost thaw [35] and/or anthropogenic land use changes like forest clear-cutting [36] or wetland drainage [37] . It should be noted that if, in contrast to our results, we assume a uniform availability for MeHg formation and bioaccumulation of the different geochemical Hg pools, the direct contributions from catchment and atmospheric pools to the total MeHg in biota are predicted to be less than 2%. The response time for MeHg concentration in fish from a changed atmospheric Hg loading rate has been predicted from experiments in lake systems to be quick in areas with mainly direct atmospheric loading, but delayed in areas dominated by catchment runoff of Hg II and MeHg [25] , [38] . Based on our results, we suggest that in estuarine ecosystems with significant catchment Hg runoff and internal MeHg production from sediment Hg II pools, reduced atmospheric Hg II loadings will only have a minor short-term effect on MeHg levels in biota and that a significant ecosystem recovery will be slow. For the type of estuarine ecosystems modelled here, a 40% decrease in global anthropogenic Hg emissions to the atmosphere (UNEPA’s postulated scenario if current emission controls planned and implemented in Europe and North America are implemented worldwide) [39] is predicted (scenario C) to only have minor short- and intermediate-term (t 0 and t R ) effects on MeHg levels in biota. A significant recovery is expected only when a reduced atmospheric Hg loading have translated into a proportional decrease in catchment MeHg and Hg II runoff. The predicted time frame to reach such conditions is highly uncertain [5] , [25] , [40] . In this paper, we present the first quantitative estimates of the contribution from different geochemical Hg pools and sources ( in situ production in sediment and input from atmosphere and terrestrial runoff) to MeHg levels in estuarine sediment and biota, taking into account both differentiated availability and size of the pools. We and others have proposed that Hg reactivity and bioavailability are controlled by combined thermodynamic and kinetic processes [14] , [19] , [41] . Thermodynamic calculations using data from the mesocosm water column ( Supplementary Table 1 ), and previous spectroscopic characterization of the Hg solid-phase speciation in the sediment used in this study [14] , show that in our experimental system reduced sulphur (organic thiols and inorganic sulphide) controls the chemical speciation of both Hg II and MeHg. We synthesized solid/adsorbed phase Hg tracers, and added them to the sediment, as defined thermodynamically favoured chemical forms (that is, β-HgS(s), Hg(SR-NOM) 2 and MeHgSR-NOM), whereas the dissolved tracers were added to the water phase as labile complexes (dominated by Hg(OH) 2 0 and MeHgOH 0 , respectively). The rationale for this approach is that the time required for Hg II and MeHg to reach equilibrium with components in the aqueous phase (including organic and inorganic particles) is relatively short (hours to maximum a few days) [18] , [19] as compared with the slower rate (days to weeks) [42] , [43] , [44] to form β-HgS(s) and adsorbed phases of Hg(SR-NOM) 2 in the sediment. As described above, the Hg II tracers added to the sediment were taken to represent sources for in situ MeHg formation and Hg II and MeHg added to the water phase were used as proxies for both terrestrial and atmospheric inputs. It should be noted that in natural environments Hg II and MeHg would be complexed mainly by thiol groups in terrestrial NOM in runoff, whereas the speciation of atmospherically derived Hg is less certain and includes dissolved inorganic Hg complexes and Hg surface complexes with organic and inorganic particles [45] . However, our state-of-the-art knowledge on Hg thermodynamics and kinetics predict that all these chemical forms would rapidly form Hg(SR-NOM) 2 and MeHgSR-NOM complexes in the oxic humic-rich brackish water of the estuary and our mesocosm systems. Previous whole-lake experiments have also indicated a rapid association of added Hg II tracers with NOM in the water column [46] . In contrast, the solid/adsorbed phase Hg tracers used in our study needed to be synthesized to thermodynamically favoured chemical forms before addition to the sediment. As illustrated in Supplementary Fig. 4, the MeHg/Hg II ratio in sediment did not vary systematically throughout the experiment for any tracer, suggesting that all tracers were already equilibrated in the system at the first measurement point at day 10. We used the MeHg/Hg II molar ratio and MeHg BSAF to quantify MeHg net formation and bioaccumulation, respectively. The calculation of relevant numbers for these parameters requires that the quantities of MeHg formed and bioaccumulated in the mesocosms are proportional to the amount of added tracer. This has been convincingly demonstrated in previous lake mesocosm experiments where the loading rate of a Hg II tracer to the water column was varied more than one order of magnitude [38] , [47] and yielded proportional amounts of formed and bioaccumulated MeHg. We used the BSAF to quantify bioaccumulation in order to facilitate a transparent comparison of accumulation of the different tracers in all the biota species (benthic invertebrates, amphipods and plankton). Further, we could only detect MeHg in the water column for the Me 199 Hg wt tracer and ambient MeHg, impeding the calculation of relevant MeHg Biota Accumulation Factor for the other tracers. Significant and fast removal of Hg tracers added to the water phase, as obtained in our systems ( Supplementary Figs 2 and 3 ), have also been observed in previous lake littoral mesocosm studies [47] , [48] . The approach we used, taking advantage of MeHg/Hg II and MeHg BSAF, rely on measured quantities of Hg II and MeHg tracers retained and circulating in the system to quantify MeHg net formation and bioaccumulation. For the ecosystem scale mass balance modelling presented in Fig. 4 we have therefore estimated the fraction of Hg influxes retained in the modelled estuary as described in the Supplementary Discussion . Similar to previous studies [47] , [49] , losses of Hg tracers from the mesocosm system is expected to occur mainly as evasion of Hg 0 (and potentially also of semivolatile MeHg complexes [50] ). Because Hg evasion was not monitored, we made no attempt to include that process in the model but relied on approaches using measured retained quantities of Hg, which are inherently independent of the magnitude of Hg losses from the system. The limitations of our experimental setup and the assumptions and associated uncertainties underlying the model parameterization are discussed in detail in the Supplementary Discussion . Sensitivity analyses of our assumptions underpinned our major conclusions in this study: that MeHg in catchment runoff loading and the solid/adsorbed phase speciation of Hg II in the sediment are the major factors controlling MeHg content in estuarine sediment and biota. To evaluate the validity and potential predictive power of the model, we compared the measured concentrations of ambient MeHg in biota collected in the mesocosm systems with modelled concentrations predicted from the MeHg/Hg II molar ratio and MeHg BSAF data generated by the added tracers and the Hg input fluxes estimated for the Öre Estuary. Using scenario A1, the ambient MeHg concentrations in plankton, amphipods and benthic invertebrates predicted by the model (1.9, 25 and 47 pmol g −1 d.w., respectively) for the Öre Estuary were in fair agreement (within a factor of 2) with the corresponding measured concentrations (2.7±1.9, 20±7.2 and 92±54 pmol g −1 d.w., respectively) of ambient MeHg in our mesocosm experiments. This agreement supports the relevance and usefulness of the key data on Hg availability for MeHg formation and bioaccumulation generated in our mesocosm study by the use of solid/adsorbed and aqueous phase Hg tracers. It has been desired [25] to predict to what extent and within what timeframe reduced anthropogenic emissions of Hg could result in considerably lower MeHg concentration in fish. Experiments have been conducted on whole-ecosystem [25] and mesocosm [38] , [40] , [47] scales where the MeHg concentration in biota has been related to increased simulated atmospheric Hg II loading rates (by addition of isotopically enriched Hg II tracers as labile complexes, presumably dominated by Hg(OH) 2 0 , to the water column). These studies consistently demonstrated that the added Hg II tracers were to a substantial extent (within days to weeks depending on system scale) methylated and incorporated in the aquatic food webs. However, the contribution to MeHg in biota was generally smaller for the added tracer compared with ambient Hg, suggesting that most biota MeHg was derived from a store of past Hg deposits [40] . Harris et al . [25] found a 30–40% increase in MeHg in fish by increasing simulated atmospheric deposition by 120% during a 3-year period in a whole-ecosystem experiment and Paterson et al . [40] found a 3–10% increase in fish MeHg as a consequence of a 200% to >400% increase in Hg II water loadings in a lake mesocosm experiment. Based on this it was predicted that reduced atmospheric Hg loadings would yield a rapid (years) initial decay in MeHg concentration in fish but that a full response would be delayed by a gradual export of Hg II and MeHg from the watershed [25] , [38] . Differences in response rate are thus expected among aquatic systems depending on the relative magnitudes of direct atmospheric Hg depositions to the water surface and Hg inputs from the watershed [25] . These studies have significantly advanced our understanding on Hg biogeochemistry, specifically on the response time of MeHg content in aquatic biota following reduced atmospheric Hg deposition. The principle experimental approach in these studies was based on comparing the fate of labile Hg II tracers added to the water phase and ambient Hg. Utilizing our new experimental approach (combining the use of Hg II and MeHg isotope tracers added to both the sediment and the water phase), we can here present novel quantitative data, not included in previous studies, on formation and bioaccumulation of MeHg from different sediment Hg pools and on differences in bioaccumulation of MeHg loadings to the water phase versus MeHg formed in situ in the sediment. One of the most striking result in our study was the considerably higher accumulation in biota of MeHg from the Me 199 Hg wt tracer compared with MeHg formed in situ in the sediment. This was observed both for benthic organisms and plankton. These results clearly emphasize the relative importance of terrestrial MeHg formation and subsequent runoff for MeHg bioaccumulation in estuarine environments. Although land runoff causes significant direct input of MeHg with high availability for bioaccumulation, Hg II from atmospheric deposition that is methylated in situ forms MeHg, which bioaccumulates to a lesser extent. It is plausible that this difference in MeHg availability would be less significant in aquatic systems with significant in situ MeHg formation in the water column [51] , and that the contribution to MeHg in biota from Hg II loadings from atmospheric depositions and land runoff would be higher in such systems. Further, our observations of high bioavailability of MeHg inputs to the water phase have largest implications for DOC-rich estuaries with a large watershed/water surface area ratio and/or large terrestrial MeHg influx rate. It can be expected that such systems will show the slowest response in MeHg levels in biota following reduced atmospheric Hg depositions. Our study also add important data to clarify the relative importance of recent atmospherically derived Hg II and accumulated Hg II pools in sediment to MeHg levels in estuarine biota [25] , [38] , [47] . Our results show that recent Hg II loadings to the water phase is more available for MeHg formation and bioaccumulation than previously deposited Hg II circulating in the ecosystem. We provide data showing that the magnitude of this discrepency, however, is largely controlled by the solid/adsorbed phase chemical speciation of Hg II in the sediment. The net MeHg formation was more than ten times higher for the 201 Hg II -NOM sed compared with the β- 200 HgS sed tracer. This suggests that the relative contribution to biota MeHg levels from the accumulated sediment Hg II pool will be much lower in systems with formation of microparticulate crystalline β-HgS. Such systems can thus be expected to exhibit a significantly stronger initial response in biota MeHg levels following reduced atmospheric Hg II deposition compared with systems dominated by Hg(SR-NOM) 2 complex formation in the sediment. Orihel et al . [48] , using an experimental approach where labile Hg II tracers were added to the water column of a lake littoral mesocosm system in two consecutive years, reported a higher MeHg concentration in plankton from the newly added tracer compared with the tracer aged for 1 year in the system. However, in a similar 2-year mesocosm Hg tracer addition experiment, Paterson et al . [40] observed the opposite trend. In view of the less available Hg II pertaining to adsorbed and solid phases in sediments reported in our study, the lower availability of Hg II tracers after 1 year of aging reported by Orihel et al . could be interpreted as an effect of HgS(s) and Hg(SR-NOM) 2 formation in sediments. Enhanced rates of MeHg formation have been observed in bacteria culture experiments amended with nanoparticulate compared with microparticulate HgS(s) [9] , [41] . The underlying mechanisms for this discrepancy, as well as the quantitative importance of nanoparticulate HgS(s) in natural sediment, however, remain unclear. If the observed differences in MeHg formation rate are due to higher solubility and/or dissolution rate of nanoparticulate HgS(s), it, if present in the sediment, may exhibit a MeHg/Hg II molar ratio in-between the observed ratios for the 201 Hg II -NOM sed and β- 201 HgS sed tracers used in our study. The recently UNEP negotiated Minamata treaty to limit anthropogenic Hg emissions [52] has further spurred questions on how fast ecosystems may recover following reduced atmospheric Hg emissions and if other changes (for example, climate) in the systems [53] can counteract or amplify the recovery processes. Such predictions have been hampered by a limited understanding on how different geochemical pools/sources of Hg in the environment contribute to MeHg in biota. Pool-specific contributions must be established to understand in detail the Hg biogeochemical cycle and for accurate predictions on the outcome of reduced anthropogenic Hg emissions and potential impacts on Hg levels in biota following climate change scenarios and anthropogenic land use. Traditional Hg mass balance models may not accurately address this issue as quantitative data on the different Hg pools’ availability to MeHg formation and bioaccumulation have been lacking. Our findings thus have far-reaching implications for central scientific questions on Hg biogeochemistry as well as applied aspects of environmental policy and should be considered in future biogeochemical Hg cycling models at regional and global scales. Site description and sampling The Öre Estuary is located at the Swedish east coast and connects to the Bothnian Sea. The estuary covers an area of 50 km 2 and has a total volume of 10 9 m 3 and average depth of 16.4 m. Öre River is the main source of suspended particles to the estuary and the bottoms are dominated by sediment with a discontinued deposition of fine grained particles (so called transportation bottoms). Intact sediment cores (~0.2 × 0.63 m 2 Ø) were manually collected by divers (coordinates: 63° 33.905′ N, 19° 50.898′ E) at water depth of 5–7 m using custom-made sampling devices consisting of HDPE (same material as the mesocosm systems described below) cylinders with detachable bottom and lid. Each cylinder was immersed into undisturbed sediment and then cleared from surrounding sediment to allow inserting the bottom plate through a notch in the cylinder wall. The lid was then placed on a rim a few centimetre above the sediment surface. The cores were lifted onto a research vessel and placed in barrels filled with brackish water to avoid leakage and direct contact with air. Sediment cores were then stored dark at 15 °C for up to 7 days. The average sediment density and dry weight were 1.18±0.03 g cm −3 and 32±4.1%, respectively. Unfiltered seawater was collected (salinity of 5 Practical Salinity Units (PSU)) using a peristaltic pump system connected to parallel pipes with the inlet located 800 m from land (in the Öre Estuary) and at water depths of 2 and 8 m. All mesocosms were filled with water in parallel to assure similar distribution of, for example, planktonic organism communities. Mesocosm system preparation and isotope tracer additions The mesocosm facility is located at the Umeå Marine Sciences Centre and consists of totally 12 double-mantled HDPE tubes (5 × 0.74 m 2 Ø) that are temperature controlled in sections via an outer layer of glycol. 150 W metal halogen lamps (MASTERColour CDM-T 150W/942 G12 1CT) were used as light source with a light/dark cycle of 12:12 h. Temperature of the water column was controlled in three sections with a set temperature of 14 °C in the top layer (0.1–1.4 m depth) and 16 °C in the middle layer (1.85–3.15 m depth) creating a mixing by thermal convection in the upper part of the water column and a thermocline at ~3.2 m between the middle and lowest section ( Supplementary Fig. 5 ). The lowest section (3.6–4.9 m depth) was set to 10 °C. Separate mesocosm experiments showed complete mixing of the upper part of the water column within a few hours. Nitrate (NO 3 − ), phosphate (PO 4 3− ) and ammonium (NH 4 + ) solutions were prepared from salts (NaNO 3 , NaH 2 PO 4 × H 2 O and NH 4 Cl) and added to the mesocosm water phase at amounts giving a concentration increase corresponding to 10% (days 1, 3, 8, 12) or 5% (days 16, 18 (only PO 4 3− and NH 4 + ), 22, 25 and 32) of the concentration typical for winter conditions in the Bothnian Sea (10 μM NO 3 − , 0.77 μM PO 4 3− , 1.8 μM NH 4 + ) [54] . The date for the first nutrient addition is referred to as day 1 and the experiment then continued for 57 days. The mesocosms were regularly filled up with fresh, tempered, brackish water (~2 l day −1 ) to compensate for losses of water from sampling and evaporation and maintain a constant water volume of ~1,950 l. Hg II enriched in 196 Hg (50%), 198 Hg (92.78%), 199 Hg (91.95%), 200 Hg (96.41%), 201 Hg (98.11%) or 204 Hg (98.11%) (as HgO or HgCl 2 ) were purchased from Oak Ridge National Laboratory. Isotopically enriched MeHg [55] and β- 200 HgS(s) [14] were synthesized as described elsewhere. The 201 Hg II -NOM and Me 198 Hg-NOM tracers were prepared according to Jonsson et al . [14] by adding 201 Hg(aq) or Me 198 Hg(aq) to a Milli-Q (MQ; resistivity >18.2 MΩ cm) water suspension of a freeze-dried and ball-milled, homogenized peat soil previously characterized by Skyllberg and Drott [56] . The estimated Hg/RSH molar ratio was kept in the range previously demonstrated to give 1:2 Hg II :RSH and 1:1 MeHg:RSH complex stoichiometry for binding of Hg to this peat soil [57] . A slurry mixture of β- 200 HgS(s), 201 Hg II -NOM and Me 198 Hg-NOM was prepared within 1 h before injected into the intact sediment cores using an electronic 12-channel pipette (VWR, 10–200 μl sample aliquots). Amounts of 12 × 100 μl of the slurry were withdrawn and injected ~0.5 cm below the sediment surface in 10 μl portions with 1 cm x axis distance (controlled using a custom made grid system) and 0.8 cm y axis distance between pipette tips, which gave 1.13 injections per cm 2 (final concentrations are given in Supplementary Table 2 ). In total, 3,264 injections were made for two of the mesocosms (denoted M2 and M3) covering 92% of the sediment surface. Owing to a disturbed surface in the outer part of the third sediment core (mesocosm denoted M1), instead 2,946 injections were made covering 83% of the surface area. Sediment not covered by tracer additions was located in the outer part of the sediment cores and no sediment sub-samples were taken from this part during the experiment. Sediment cores were spiked and immersed into water-filled mesocosms with the lid removed after placement of the sediment cylinders on bottom of the mesocosm tubes to protect the sediment surface during placement. 204 Hg II wt and Me 199 Hg wt were added day 2 of the experiment to the upper part of the water column (above the thermocline) 20 min after light was turned off, that is, at the beginning of a 12-h dark cycle to minimize evasion losses [49] . Sampling and analysis Water and sediment were sampled once a week from the mesocosms for the determination of primary and bacterial production rates ( Supplementary Fig. 6 ), DOC, humic matter, light transmittance and O 2 saturation ( Supplementary Table 3 ) and Hg II methylation and MeHg demethylation rate constants ( k m and k d (d −1 )), and concentrations of nutrients, Chl α, total Hg (tot-Hg) and MeHg in water as well as determination of k m and k d , dry weight and the concentrations of MeHg and tot-Hg in sediment. Sediment sub-cores were sampled from the mesocosm sediments during the experiment using a custom-made sampler designed for the mesocosms ( Supplementary Fig. 7 ). Depth profiles of H 2 S, O 2 , redox and pH were also measured in sediment samples using microelectrodes (Unisense). Sedimented material was collected for determination of δ 13 C, δ 15 N, C (%) and N (%) and the concentrations of MeHg and tot-Hg. Seston size fractions and benthic organisms were collected at the end of the experiment for determination of δ 13 C, δ 15 N, C (%) and N (%) and concentration of MeHg and tot-Hg. Pressure, turbidity and O 2 were measured in situ in the water column using a Seaguard CTD with attached microelectrode sensors (Unisence) and light penetration using a Spherical Quantum Sensor (LI-COR, 193-SA and LI-COR 1400 unit). Details of sampling and analysis are provided in the supporting information. Briefly, the concentratons of tot-Hg and MeHg in water, sediment and biota were determined using 196 Hg II or Me 196 Hg as internal standard for isotope dilution analysis, matrix and analyte-specific extraction and preconcentraiton techniques followed by inductively coupled plasma mass spectrometry (ICPMS) analysis for tot-Hg and Gas Chromatography-ICPMS analysis for MeHg. Concentrations of tot-Hg and MeHg for ambient Hg and tracers were then calculated from mass-bias corrected signals using signal deconvolution [58] . The determined Hg parameters and concentrations are given in Supplementary Tables 4–8 . Detection limit and quality control for Hg determinations With the experimental setup in this study, the signals for individual Hg isotope tracers in the ICPMS analyses are detected superimposed on a ‘background’ of ambient Hg and contributions from minor isotopes of the other tracers present in the sample. The limit of detection (LOD) can therefore not be assessed by common approaches with blank samples. Indeed, the LOD for tot-Hg and MeHg determinations will vary among individual tracers and samples. We defined LOD for Hg tracers as the Hg amount giving a 4.8% signal contribution to the total measured signal intensity at the specific isotope mass. This factor was determined based on typical expanded uncertainties in measured signal intensities, and thus an individual LOD was calculated for each isotope tracer and sample. Certified reference materials were analysed with every sample batch for the determination of MeHg and tot-Hg concentrations in sediment and biota. The obtained results (average±CI, P =0.05) were 81±2 ng MeHg per g d.w. ( n =33) for MeHg in sediment (ERM-CC580, certified value 75±4 ng MeHg per g d.w.), 683±39 ng Hg per g d.w. ( n =4) for MeHg in biota (DOLT-2, certified value 693±53 ng Hg per g d.w.), 102±6 ng Hg per g d.w. ( n =6) for tot-Hg in sediment (Mess-3, certified value 91±9 ng Hg per g d.w.) and 2.24±0.08 μg Hg per g d.w. ( n =8) for tot-Hg in biota (DOLT-2, certified value 2.14±0.28 μg Hg per g d.w.). Well-established standard procedures were used for all other determined parameters. Hg mass balance model We calculated the concentration of ambient MeHg in sediment and biota using equations (1) and (2), respectively. Scenario A1 and A2 were based on estimated present day catchment runoff and atmospheric deposition inputs of Hg II and MeHg to the Öre Estuary. Amounts of accumulated Hg II in the sediment present as β-HgS(s) and Hg II -NOM, respectively, were calculated from an average concentration of ambient tot-Hg (280 pmol g −1 d.w.) for five sampling sites within the estuary estimated from data reported by Lambertsson and Nilsson [27] , and a β-HgS(s)/Hg II -NOM molar ratio of 70:30 in scenario A1 (as determined previously for sediments from the same sampling location using L III -edge Hg-EXAFS [14] ) and 30:70 in scenario A2. In scenario B, we modelled a two times increase in catchment runoff loading of Hg II and MeHg, and in scenario C, we modelled a 40% reduction in anthropogenic atmospheric emission of Hg (as predicted by Pacyna et al . [39] , [59] for 2020 if emission controls planned and implemented in Europe and North America are implemented worldwide) resulting in a net decrease of total atmospheric Hg II deposition of 27% (assuming that 67% of the total amount of atmospheric Hg emissions are anthropogenic [60] ). The total MeHg concentration in sediment ([MeHg] sed ; pmol g −1 d.w. in 0–1.5 cm) and specific contributions from different geochemical Hg pools were calculated using MeHg/Hg II molar ratios determined from isotope-enriched Hg II and MeHg tracers in the mesocosm experiment, estimated loading rates of Hg II and MeHg from catchment runoff and atmospheric deposition (mol per 4 months; Table 1 ) and Hg II and MeHg stored in the top 1.5 cm of the sediment as β-HgS(s) and Hg II -NOM (mol). MeHg stored in sediment and not readily available for demethylation was calculated using a factor, F [MeHg]sediment , set to 0.30 of the sum of the other contributing sources. The absolute amounts of MeHg (mol in 0–1.5 cm) were recalculated to a concentration (pmol g −1 d.w. in 0–1.5 cm) using a conversion factor C of 3.53 × 10 12 g −1 d.w. ( C =(density sed (g w.w. cm −3 ) × d.w./wet weight (w.w.) ratio × sediment depth (cm) × estuary area (cm 2 )) −1 × 10 12 ). The total MeHg concentration (pmol g −1 d.w.) in biota ([MeHg] biota ) and specific contributions from different geochemical Hg pools were calculated using the predicted concentration of MeHg (pmol g −1 d.w.) in the sediment (0–1.5 cm) from each geochemical Hg pool calculated by equation (1) (for example, as ) and BSAF determined using isotope enriched Hg II and MeHg tracers in the mesocosm experiment, where, for example, denotes BSAF for MeHg formed from the 204 Hg II wt tracer. Statistical data treatment All data are presented as average±CI ( p =0.05). Differences in MeHg/Hg II molar ratios and MeHg BSAFs of isotopically enriched tracers and ambient Hg were tested by one-way analysis of variance ( Supplementary Tables 4 and 5 , with their underlying raw data given in Supplementary Tables 6–8 ). If α <0.05 the null-hypothesis (no difference among treatments) was rejected and Tukey’s post hoc analysis ( p =0.05) was used to identifying groups statistically differing. All calculations were conducted using EXCEL 2010 (Microsoft). How to cite this article: Jonsson, S. et al . Differentiated availability of geochemical mercury pools controls methylmercury levels in estuarine sediment and biota. Nat. Commun. 5:4624 doi: 10.1038/ncomms5624 (2014).